Observation of correlated spin–orbit order in a strongly anisotropic quantum wire system Quantum wires with spin–orbit coupling provide a unique opportunity to simultaneously control the coupling strength and the screened Coulomb interactions where new exotic phases of matter can be explored. Here we report on the observation of an exotic spin–orbit density wave in Pb-atomic wires on Si(557) surfaces by mapping out the evolution of the modulated spin-texture at various conditions with spin- and angle-resolved photoelectron spectroscopy. The results are independently quantified by surface transport measurements. The spin polarization, coherence length, spin dephasing rate and the associated quasiparticle gap decrease simultaneously as the screened Coulomb interaction decreases with increasing excess coverage, providing a new mechanism for generating and manipulating a spin–orbit entanglement effect via electronic interaction. Despite clear evidence of spontaneous spin-rotation symmetry breaking and modulation of spin-momentum structure as a function of excess coverage, the average spin polarization over the Brillouin zone vanishes, indicating that time-reversal symmetry is intact as theoretically predicted. The spin degree of freedom of electrons has attracted much attention over the last several years and plays a central role in spintronic device structures [1] , the spin Hall effect [2] , [3] , topological insulators [4] , Rashba-type surface or interface states [5] , [6] and others. Typically, the propagation of electrons is treated as a single-particle problem. This simple concept fails, however, when electronic correlation effects become important and spin- and orbit effects are entangled such as in hard magnets (ref. 7 ), j =1/2 Mott insulators [8] or in new emergent topological superconductors [9] , [10] , [11] . Among others, the spin-ordered Au-chain ensemble grown on Si(553) (refs 12 , 13 , 14 ) and also magnetic chain structures on insulating or superconducting surfaces [15] , [16] , [17] are recent illustrations of this entanglement and have attracted a lot of research activities owing to their full flexibility for manipulation with atomic precision. Reminiscent of antiferromagnetism in Cr [18] , the problem of spin–orbit coupling (SOC) under consideration of electronic interaction has been revisited recently [11] , [19] . It was shown that inherent spin splitting such as Rashba-type SOC yields Fermi surfaces (FS) with nesting between opposite helical states causing a so-called spin–orbit density wave (SODW) state which cannot be characterized by independent local order parameters. This new emergent phase of matter arises without breaking time-reversal symmetry above a critical value for the Coulomb potential U and its order parameter, i.e. the energy gap Δ, is determined by the energy scales of both the SOC strength λ and the interaction U [19] . Furthermore, a finite gap Δ protects the SODW from spin dephasing against external perturbations like magnetic fields, thermal excitation and doping by excess coverage. In case that the interaction energy is large compared to the SOC, however, the SODW can be overturned at the expense of a spin density wave. Experimentally, a SODW can be identified by the difference between charge and spin order, the nesting of spin-polarized states and the concomitant opening of a gap, and the depolarization of the spin order as a function of Coulomb screening due to the dephasing of spin states. The observation of all these signatures in our experimental data will be addressed subsequently after a brief introduction into our quantum wire system of choice, that is, epitaxially grown Pb wires on Si(557) (refs 20 , 21 , 22 ). Most remarkably, at the critical concentration of 1.31 monolayers (ML), a one-dimensional (1D) gap Δ=20 meV is opened below 78 K so that the Pb layer becomes insulating in the direction perpendicular to the wires while it remains conducting along the chain direction [23] , [24] . As sketched in Fig. 1b , this bandgap opening is caused by Pb-induced refacetting of the (557) orientation to (223)-oriented facets, thus introducing a new reciprocal lattice vector, g =2 πd −1 e , which fulfils the (spin-polarized) nesting condition 2 k F = g along the direction, which is one of the signatures for the formation of a SODW as discussed above ( d is the interwire distance, k F is the Fermi wave vector and e is the unit vector). This condition is superimposed on the local two-dimensional (2D) character of the densely packed phase of Pb on the mini-(111) terraces, which is reflected by closed Fermi circles rather than by open Fermi lines ( Fig. 1c ). The Fermi nesting in this system leads to the expected renormalization of the FS [24] . For the sake of simplicity and the fact that the gap is comparably small, we show here the quasi-FS, that is, the circularly shaped spectroscopic features seen at E F —50 meV. This representation takes also the replica bands into account that are seen by the momentum distribution curves (MDCs) taken necessarily also slightly below E F . A large degree of geometrical order along the wires, coupled with high 1D conductance, is evident by the 10-fold superperiodicity ( s =10 × a Si ) at the critical coverage of 1.31 ML, shown by high-resolution scanning tunnelling microscopy (STM) in Fig. 1a and also seen by spot splitting in low-energy electron diffraction (LEED, see below). Strikingly, the system reveals giant Rashba splitting of Δ k 0 =0.2 Å −1 (Rashba parameter α R =1.9 eV Å; ref. 25 ), which is by far larger than the expected value for chemisorbed Pb ML on isotropic semiconducting surfaces, for example, Pb/Ge(111) (ref. 26 ). Δ k 0 corresponds to exactly g / 2 , that is, the periodicity of spin ordering is twice than that of charge ordering at this critical Pb concentration, so that spins on adjacent terraces are coupled in an anti-parallel manner. This spin-dependent splitting is marked in Fig. 1b,c by different colours. The different periodicities of spin and charge are a necessary prerequisite for non-trivial coupling between them. 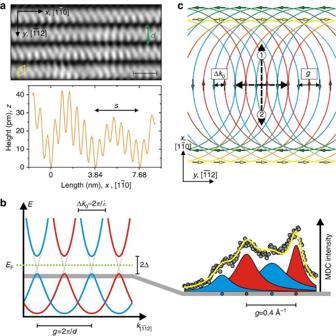Figure 1: Atomic and electronic structure of quantum wire ensemble. (a) STM (+1 V) revealing the interwire spacingd=1.58 nm of a (223) facet structure (scale bar, 2 nm). The period ofcorrelates with formation of a Pb-reconstruction (yellow trapeze shows size of the unit cell). The superimposed modulation ofs=10 ×aSiis seen as a spot splitting in the LEED patterns inFig. 2as well. (b) Schematic of the band structure in the direction across the wires (direction). The two colours denote the spin orientation in each of the subbands. The distance between bands with thesamespin helicity isg=2π/d=0.4 Å−1. The Fermi nesting driven energy gap Δ=20 meV has been determined by ARPES and transport measurements23,24,33. Right: the equidistant sequence of both spin bands is nicely reflected by the MDC (spin-integrated) taken at the valence band maximum along thedirection. The spin signature of the subbands has been deduced from spin-resolved measurements25. (c) The giant SOC ensures a constructive interference of FS with the same helicity in k-space along thedirection. Renormalization of the FS gives rise to a ‘hotspot’ wave vectorΔk0. The direction along the wires is discussed in context withFig. 4a–c. Figure 1: Atomic and electronic structure of quantum wire ensemble. ( a ) STM (+1 V) revealing the interwire spacing d =1.58 nm of a (223) facet structure (scale bar, 2 nm). The period of correlates with formation of a Pb- reconstruction (yellow trapeze shows size of the unit cell). The superimposed modulation of s =10 × a Si is seen as a spot splitting in the LEED patterns in Fig. 2 as well. ( b ) Schematic of the band structure in the direction across the wires ( direction). The two colours denote the spin orientation in each of the subbands. The distance between bands with the same spin helicity is g =2 π/d =0.4 Å −1 . The Fermi nesting driven energy gap Δ=20 meV has been determined by ARPES and transport measurements [23] , [24] , [33] . Right: the equidistant sequence of both spin bands is nicely reflected by the MDC (spin-integrated) taken at the valence band maximum along the direction. The spin signature of the subbands has been deduced from spin-resolved measurements [25] . ( c ) The giant SOC ensures a constructive interference of FS with the same helicity in k-space along the direction. Renormalization of the FS gives rise to a ‘hotspot’ wave vector Δ k 0 . The direction along the wires is discussed in context with Fig. 4a–c . Full size image Here we show that in this array of atomic wires bound to the (223)-oriented facets on Si(557), we have the unique possibility to tailor the interwire coupling by adsorption of minute amounts of excess coverage δ Θ. The screened Coulomb potential scales with the size of the excess coverage as U ( δ Θ)= U (0)·exp(− qδ Θ), where q is the screening parameter [27] . As we will show, while the spin–orbit order is preserved (at least) up to a critical additional coverage of 0.1 ML, steps are decorated by this excess coverage not randomly, but by formation of superstructures whose periodicity depends on excess concentration of Pb [20] , [28] . This highlights that the mechanisms of spin and charge order are not the same. The coupling between charge and spin order is mediated by 1D in-gap states and is reduced with increasing excess coverage. This leads to spin depolarization as a function of excess coverage. Therefore, this mechanism has much more fundamental consequences than the band shift associated with standard doping, an observation that has been made also in other metallic chain systems on surfaces [29] , [30] , however, with somewhat different physical scenarios. A collapse of the SODW phase is associated by an almost vanishing spin polarization close to δ Θ≈0.2 ML, where the Pb wires turn into an anisotropic 2D metal. Quite naturally, SODW formation and the reduced spin–charge coupling as a function of excess Pb concentration also influence other physical properties that are sensitive to both charge and spin, such as magnetotransport. As expected, the gradual spin depolarization seen in photoemission is closely related to the spin dephasing probed by magnetotransport measurements [31] . This relationship can be quantitatively described by SODW theory, as we will demonstrate below. The effect of excess coverage Adsorption of excess coverage on the perfect Pb-chain system, as shown in Fig. 1a , changes primarily the periodicities of the Si(557) surface perpendicular to the wires. We demonstrate by the results collected in Fig. 2 that spin and geometric order indeed do not have the same periodicities, although they are connected and commensurate to each other by the underlying terrace structure. Moreover, while the charge order follows the geometry, the spin order turns out to be robust and unchanged by excess coverage. 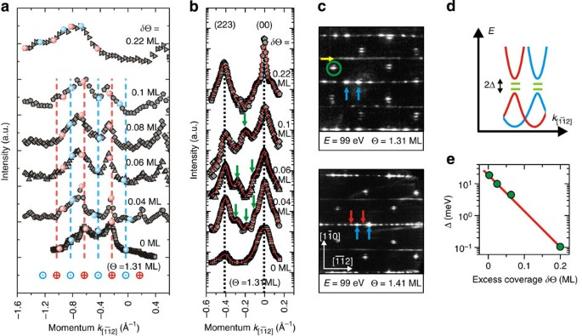Figure 2: Evolution of wire structure with additional coverage. (a) Sequence of the spin-integrated MDCs taken along thedirection for various excess coveragesδΘ. The symbols denote the spin texture and have been deduced from spin-resolved measurements (Supplementary Fig. 1). To reveal good signal/noise ratios in reasonable time, the spin distribution has been measured 50 meV below the Fermi level. (b) LEED diffraction profiles alongdirection of the 1.31 ML Pb/Si(557) phase with variousδΘ. Formation of long-range-ordered chains are marked by arrows. (c) 2D LEED pattern withδΘ=0 ML andδΘ=0.1 ML. The latter shows nicely the doubling of the period along thedirection (red arrows)28. Optical LEED patterns are shown in theSupplementary Note 2. (d) Schematic showing the appearance of new in-gap states. (e) The gradual decrease of the bandgap Δ with increasingδΘ deduced from a previous transport measurement27. The error bars deduced from the transport experiments are around 10%. The (red) regression line follows Δ=20 meV·exp(−δΘ/0.038 ML). Figure 2: Evolution of wire structure with additional coverage. ( a ) Sequence of the spin-integrated MDCs taken along the direction for various excess coverages δ Θ. The symbols denote the spin texture and have been deduced from spin-resolved measurements ( Supplementary Fig. 1 ). To reveal good signal/noise ratios in reasonable time, the spin distribution has been measured 50 meV below the Fermi level. ( b ) LEED diffraction profiles along direction of the 1.31 ML Pb/Si(557) phase with various δ Θ. Formation of long-range-ordered chains are marked by arrows. ( c ) 2D LEED pattern with δ Θ=0 ML and δ Θ=0.1 ML. The latter shows nicely the doubling of the period along the direction (red arrows) [28] . Optical LEED patterns are shown in the Supplementary Note 2 . ( d ) Schematic showing the appearance of new in-gap states. ( e ) The gradual decrease of the bandgap Δ with increasing δ Θ deduced from a previous transport measurement [27] . The error bars deduced from the transport experiments are around 10%. The (red) regression line follows Δ=20 meV·exp(− δ Θ/0.038 ML). Full size image The respective charge and spin order can be seen in Fig. 2a , which shows the electronic structure perpendicular to the wires. Here the periodicity of the facet structure is seen in spectroscopy by Umklapp scattering. From the intense MDC peak structure of the perfect wire ensemble ( Fig. 1b ), a modulation vector of 0.4 Å −1 can be deduced in agreement with the spot splitting along the direction visible in LEED. However, as mentioned before, the MDC signal reveals an additional substructure, which is shifted by 0.2 Å −1 and has the opposite spin helicity [25] . In Fig. 2a , we marked the extrema of the x -component of the spin polarization by red- and blue-coloured circles. This equidistant splitting is a spectroscopic hallmark for a SODW in its ground state [19] . Note that we present throughout the paper spin-integrated MDCs measured with high resolution. The colour-coded spin components shown are deduced from additional MDCs recorded with the Mott detector ( Supplementary Note 1 and Supplementary Fig. 1 ). To reveal good signal/noise ratios in reasonable time, the spin distribution has been measured 50 meV below the Fermi level. However, the excellent agreement with results from direct current (DC)- and magnetotransport demonstrate that this limitation does not affect our conclusions at all. With increasing δ Θ, we see that the intensities in the MDCs are slightly altered due to changing photoelectron scattering conditions related to the geometrical superperiodicities (see below). However, and more importantly, the positions of the maxima of spin polarization remain unchanged in k-space. In contrast to the geometric order, the original spin periodicity found at δ Θ=0 ML of 0.2 and 0.4 Å −1 , respectively, prevails until we reach the limit of second Pb layer growth at an excess coverage of 0.2 ML. At this excess coverage also the original SODW phase collapses, as seen by negligible spin polarization of all three components. Since the enhanced spin-texture along the FS nesting direction only appears below 0.2 ML excess coverage and below 78 K, it strongly indicates to be an interaction effect, rather than a single-particle SOC effect. We therefore conclude that the periodicity of spin order up to δ Θ=0.2 ML is exclusively determined by the periodicity of the terrace structure of (223) facets. This terrace-induced spin order is reached with maximum spin polarization at the critical concentration of Θ=1.31 ML, and is interpreted to represent the ground state of the SODW. Looking at the geometric order, the diffraction pattern of the perfect phase ( δ Θ=0 ML; Fig. 2c ) reveals several characteristic features, for example, pronounced facet spots along (blue arrows), spots (green circle) and intensity streaks at × 2 positions (yellow arrows), originating from the long-range-ordered (223) facet structure (step density 21%), densely packed Pb reconstruction on the (111) units and Si-dimerization taking place at step sites, respectively. In high-resolution LEED studies, the spots show splitting of 2 π / s =0.16 Å −1 due to formation of domain walls giving rise to 10-fold periodicity ( s =38.4 Å) along the wires [20] , [28] , as confirmed by our STM study ( Fig. 1a , Supplementary Note 2 , and Supplementary Figs 4 and 5 ). Similar observations were made for Pb/Si(553) (ref. 32 ). On deposition of excess coverage, superstructure spots appear within the initial diffraction pattern of the 1.31 ML phase whose periodicity is reduced by integer multiples of the terrace lattice constant as a function of δ Θ (see diffraction line profiles perpendicular to the steps plotted in Fig. 2b ). As an example, for δ Θ=0.1 ML, the periodicity along the direction is doubled (see red arrows) by decoration of every second terrace [28] . This variation of geometric order induced by excess coverage is coupled with the reduction of the bandgap, as measured previously [27] . The results, reproduced in Fig. 2e show that subbands are formed within the bandgap (see schematic of Fig. 2d ), which gradually fill the gap as a function of δ Θ. The gradual decrease of the bandgap follows Δ=20 meV· exp(− δ Θ/0.038 ML), which corresponds to q =26.3 per ML. Regarding the influence of geometric periodicities on the spin order observed, there is obviously no direct impact of the modified chain structures, but the (223) structure is still observed in LEED at all excess coverages and at low temperature (cf. Fig. 2b ). This is the only geometric feature remaining constant on adsorption of excess coverage. Therefore, coupling between spins on adjacent terraces can only be mediated via the bandgap. Consequently, the reduction of the bandgap also reduces the effective coupling between spin order on different terraces. In other words, decoration of the step edges with various periodicities and excess coverages increases the screened Coulomb interaction, which couples to spin order via spin–orbit interaction. This is exactly the SODW scenario. Spin dephasing in ARPES Whether this concept holds can be tested by looking at excitations of the ground state represented by the spin order at the critical Pb concentration of 1.31 ML. Regardless of the protection of the SODW phase, the spin polarization of the surface bands should be affected by the excess coverage since the spin dephasing time is proportional to the size of the electronic gap [19] . 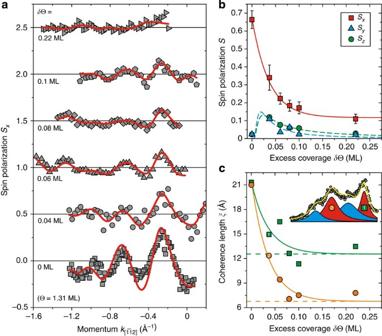Figure 3: Damping of spin polarization and coherence length. (a) Spin polarization along the wires measured along thedirection for different amounts of excess coverage. The spectra are shifted for better visibility (Sy-,Sz-components and Mott MDCs are shown in theSupplementary Fig. 2). (b) Peak-to-peak maximum values of all three polarization vectors as a function of excess coverage. The (solid) line is deduced from theory. The dashed lines are guide to the eyes. The error bars are deduced from least mean square fits to the spin-polarized ARPES data. (c) Coherence lengthsξ=2/FWHM deduced from the FWHM (after deconvoluting the spectrometer function) of the two most intense peaks of the Mott MDCs. The data point for the clean system was recalculated from spectra taken atT=60 K. Figure 3a shows S x -polarization curves obtained along the direction, revealing a pronounced spin polarization along the wires ( direction). Up to δ Θ=0.1 ML the polarization curves reveal an harmonic but damped oscillatory behaviour. The period of 0.4 Å −1 as well as the almost symmetric amplitudes, is giving rise to a vanishing net polarization within the Brillouin zone ( P =0), indicating the presence of time-reversal symmetry. This observation excludes the possibility of a spin density wave and further favours the SODW scenario [19] . Figure 3: Damping of spin polarization and coherence length. ( a ) Spin polarization along the wires measured along the direction for different amounts of excess coverage. The spectra are shifted for better visibility ( S y -, S z -components and Mott MDCs are shown in the Supplementary Fig. 2 ). ( b ) Peak-to-peak maximum values of all three polarization vectors as a function of excess coverage. The (solid) line is deduced from theory. The dashed lines are guide to the eyes. The error bars are deduced from least mean square fits to the spin-polarized ARPES data. ( c ) Coherence lengths ξ =2/FWHM deduced from the FWHM (after deconvoluting the spectrometer function) of the two most intense peaks of the Mott MDCs. The data point for the clean system was recalculated from spectra taken at T =60 K. Full size image To quantify the spin depolarization, we have plotted the peak-to-peak values of the most intense oscillations for all three spin components ( Fig. 3b ). The S x -component decreases exponentially with increasing excess coverage and can be well described by S x ( δ Θ)=0.56·exp(− δ Θ/0.036 ML)+0.12, that is, q =27.8 per ML. The (solid) line is a fit according to the SODW theory (see below). We want to emphasize that the gradual decrease of the bandgap Δ deduced independently from DC-transport measurements reveals an almost identical q value. As shown in Fig. 3b , the S y - and S z - components are considerably weaker ( Supplementary Fig. 2 ). For an ideal Rashba system, these components should vanish, while in presence of excess coverage this rule is lifted and might be indicative of spin spirals [11] . After the bandgap has vanished a fast dephasing of the spin-polarized photoholes within the SODW state mimics almost unpolarized surface bands. As expected, the effect of depolarization comes along with a reduction of the coherence length ξ . Figure 3c shows ξ of the photoelectrons deduced from the full-width of half-maximum (FWHM)=2 ξ −1 for two MDC peaks as a function of excess coverage which follow a similar trend as the spin polarization. Moreover, the spin texture along the wires for the quasi-perfect structure has also been measured. As obvious from the MDC shown in Fig. 4b , the most intense features stem from Fermi circles around —points of adjacent Brillouin zones and their replicas as depicted by the corresponding labels in Fig. 4c . In agreement with the analysis of transport presented below, only the central part of the momentum space is relevant. The 2 π / s modulation reflecting the domain wall configuration along the wires (cf. ref. 24 ) is seen mainly by further satellite peaks shown in Fig. 4b . Only their consideration allows a comprehensive description of the spin polarizations and corresponding Mott MDCs ( Fig. 4a ). At least for the S x - and S y -components significant spin signals are found. Most importantly, the spin signal around k ≈0 Å −1 reveals only a single-spin component giving rise to a spin-polarized transport channel as we will show below ( S z -component shown in Supplementary Fig. 3 ; ref. 33 ). 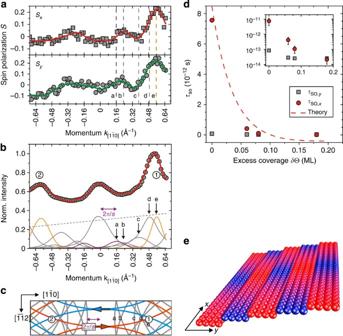Figure 4: Spin structure along the wires and SODW. (a)Sx- andSy-components along thedirection (Szis shown inSupplementary Fig. 3). (b) MDC taken along the direction of the wires without excess coverage. The peak aroundk≈0 has a fixed spin polarization. (c) Quasi-FS including replica bands from all-points. The labels refer to those shown inaandb, andFig. 1c. The 10-fold periodicity correlates with the replicas along thedirection. (d) Spin–orbit scattering times as a function of excess coverage deduced from magnetotransport measurements31. The dashed line is a fit according SODW theory forτSO,x, that is, along the wires. For reference also the scattering timeτSO,yfor direction across the wires is shown. Inset: log scale. (e) Real space sketch of antiferromagnetically coupled spin spirals (y-direction) propagating along the wires (x-direction). For the sake of simplicity, the 10-fold periodicity is not shown. Figure 4: Spin structure along the wires and SODW. ( a ) S x - and S y -components along the direction ( S z is shown in Supplementary Fig. 3 ). ( b ) MDC taken along the direction of the wires without excess coverage. The peak around k ≈0 has a fixed spin polarization. ( c ) Quasi-FS including replica bands from all -points. The labels refer to those shown in a and b , and Fig. 1c . The 10-fold periodicity correlates with the replicas along the direction. ( d ) Spin–orbit scattering times as a function of excess coverage deduced from magnetotransport measurements [31] . The dashed line is a fit according SODW theory for τ SO, x , that is, along the wires. For reference also the scattering time τ SO, y for direction across the wires is shown. Inset: log scale. ( e ) Real space sketch of antiferromagnetically coupled spin spirals ( y -direction) propagating along the wires ( x -direction). For the sake of simplicity, the 10-fold periodicity is not shown. Full size image Surface magnetotransport The dephasing behaviour can also be derived from magneto conductance, mainly stemming from the electronic states at E F (ref. 31 ). The scattering times for various amounts of excess coverage have been determined from a Hikami analysis [34] of the magnetotransport data and are plotted in Fig. 4d (for further details, see Supplementary Note 3 and Supplementary Fig. 6 ). In context of the depolarization presented above, the spin–orbit scattering time τ SO is of particular interest. As obvious from Fig. 4d , the spin–orbit scattering rate deduced for the direction ( x , along the wires) depends crucially on the amount of excess coverage. The strong suppression of spin–orbit scattering in absence of any excess coverage is reminiscent of spin-polarized transport along the wires. Furthermore, the spin–orbit scattering rate is reduced by at least two orders of magnitude on deposition of excess coverage, and reveals a close correlation with the depolarization and decoherence behaviour seen in angle-resolved photoemission spectroscopy (ARPES). We want to point out that this is per se not self-evident because ARPES and transport probe electrons at different energies. Regardless, it is remarkable that the spin polarization follows the same trend, which in turn demonstrates the close entanglement of both quantities and is a hallmark of strong electronic correlation. As we will show below, both can be consistently explained in terms of the SODW formalism. Based on our findings and the fact that within first order the spin lifetime τ s is given by the spin–orbit scattering time τ SO in a strongly spin–orbit-coupled system, the spin dynamics can be described by a kinetic equation [35] : where S k is the spin polarization vector, P is any external spin source and η is the scattering time. Ω k is the effective Larmor frequency defined in our case by Ω k =(Ω R k x / k F ,0,Ω SODW ), where Ω R =2 α R k F / ħ , and Ω SODW =2Δ/ ħ are the frequencies corresponding to Rashba-type SOC and SODW, respectively. In our case, P =0, and the initial condition for the spin is S k (0) x (the other components of the spin polarization are negligibly small), so we can solve the above equation analytically in the limit of Ω R <Ω SODW at the Fermi momentum, and get S x ( t )= S x (0)· exp(− t / τ so ), where the spin dephasing time is (see for details Supplementary Note 4 ) Inserting the exponential dependence of the SODW gap on the excess coverage and keeping all other parameters constant, we get a good fit of the spin dephasing time τ so to the experimental value for a reasonable parameter set of SODW gap Δ=20 meV, η =1 × 10 −12 s and Ω R =2.6 × 10 12 Hz, which is small compared with Ω SODW up to δ Θ=0.1 ML. Using the value of α R =1.9 eV Å as the Rashba parameter found in our previous study [25] , this refers to an extremely small Fermi wave vector component along the wires ( k F, x ≈10 −4 Å −1 ). This in turn explains the insensitivity of the propagating electrons along the wires against atomic-sized defects [23] . Focusing on the direction along the wires, the emergent modulated spin texture in real space can be described by dynamic spin spirals that are antiferromagnetically coupled between the wires as illustrated in Fig. 4e . The antiferromagnetic coupling along the direction is a consequence of the helical nesting found in ARPES [25] . The spin texture along the direction of wires represents the dynamic analogue to static 1D skyrmions as observed by STM in magnetic structures [36] , [37] . Our results are representative for systems where SOC and electron correlations are of comparable strength and with a negative exchange coupling. While the SODW is robust and insensitive to these couplings, the spin polarization is strongly affected and only in the pure SODW phase highly spin-polarized transport can be expected. In this respect, the continuous improvement in the field of ultra-high spin-resolved spectroscopy will allow us to investigate this new quantum phase and the associated bandgap at soonest in more detail [38] , [39] . Our investigations have further shown that the electrons within the SODW phase are strongly correlated with electrons residing as gap states. With a large screened interaction by reducing the excess coverage, the electronic states also become insulating, opening up a possibility for the realization of SODW order induced Luttinger liquid in quantum wires. Sample preparation and measurements Spin- and angle-resolved photoemission measurements have been performed at the COmplete PHotoEmission Experiment (COPHEE) end station at the Surface and Interface Spectroscopy (SIS) beamline of the Swiss Light Source [40] . The data were analysed as described in ref. 41 . Atomic wire structures were grown by evaporation of Pb on Si(557) substrates. The Pb evaporator used in this study has been calibrated before with an accuracy of 0.01 ML by analysing numerous so-called Devil’s staircase phases on Si(111) (1 ML=7.83 × 10 14 atoms per cm 2 ; ref. 42 ). The morphology of the clean Si(557) substrate as well as the structure of the wire ensemble has been checked by LEED (see Supplementary Note 2 ). Details about the preparation and coverage calibration are reported elsewhere [24] . All photoemission experiments were performed with p-polarized light with a photon energy hv =24 eV at a base pressure of 1 × 10 −8 Pa. By recording intensities and spin-induced scattering asymmetries with the two orthogonal Mott detectors for different emission angles, spin-resolved MDCs close to the Fermi energy have been measured. To reveal good signal/noise ratios in reasonable time, the spin distribution has been measured 50 meV below the Fermi level. Nearly all ARPES measurements have been performed at T =25 K while the excess coverage was deposited during the cooling phase at 80±10K. Further details about ARPES, STM and the surface (magneto) transport are reported in the Supplementary Notes 1–3 . How to cite this article: Brand, C. et al. Observation of correlated spin–orbit order in a strongly anisotropic quantum wire system. Nat. Commun. 6:8118 doi: 10.1038/ncomms9118 (2015).